Exceptional fossil preservation demonstrates a new mode of axial skeleton elongation in early ray-finned fishes Elongate body plans have evolved independently multiple times in vertebrates, and involve either an increase in the number or in the length of the vertebrae. Here, we describe a new mechanism of body elongation in saurichthyids, an extinct group of elongate early ray-finned fishes. The rare preservation of soft tissue in a specimen of Saurichthys curionii from the Middle Triassic (Ladinian) of Switzerland provides significant new information on the relationship between the musculature and the skeleton. This new fossil material shows that elongation in these fishes results from doubling the number of neural arch-like elements per myomeric segment. This unique way of generating an elongate body plan demonstrates the evolutionary lability of the vertebral column in non-teleostean fishes. The shape and arrangement of preserved myosepta suggest that S. curionii was not a highly flexible fish, in spite of the increase in the number of neural arch-like elements. Elongation of the body has evolved multiple times among vertebrates, as exemplified by snakes and numerous other groups of reptiles, as well as amphibians, mammals and fishes [1] , [2] , [3] . Changes in the axial skeleton drive that process in most cases, either through elongation or addition of vertebrae [1] , [2] , [3] , [4] , [5] ( Fig. 1 ). These changes are easily linked to changes in embryonic patterning, as a 1:1 relationship between the number of vertebrae and the number of embryonic somites [5] , [6] generally holds true in amniotes [7] as well as in ray-finned fishes [8] , [9] , and permits palaeontological data to be included when considering the developmental bases of body elongation. 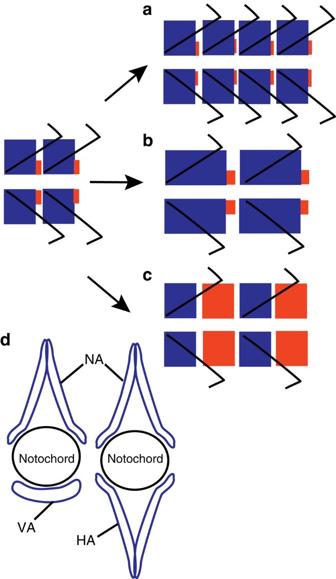Figure 1: Mechanisms of axial elongation in fishes. (a) Addition of segments, (b) elongation of segments and (c) expansion of intercalaries in lateral view. (d) Relationship between the neural and haemal arches and the notochord in anterior view. Blue represents the neural and haemal arches, red represents the intercalaries, black lines illustrate the epaxial and hypaxial myosepta. HA, haemal arch; NA, neural arch; and VA, ventral arch. Figure 1: Mechanisms of axial elongation in fishes. ( a ) Addition of segments, ( b ) elongation of segments and ( c ) expansion of intercalaries in lateral view. ( d ) Relationship between the neural and haemal arches and the notochord in anterior view. Blue represents the neural and haemal arches, red represents the intercalaries, black lines illustrate the epaxial and hypaxial myosepta. HA, haemal arch; NA, neural arch; and VA, ventral arch. Full size image In fishes, body elongation is related to the evolution of both an eel-like and an ‘ambush-predator’-type body plan [5] , one of the extremes of the large morphospace occupation that characterizes the largest radiation of living vertebrates. Specializations of this kind appeared early in the evolutionary history of ray-finned (actinopterygian) fishes [10] , [11] , with the latter body plan first becoming common in saurichthyids, a non-teleostean clade from the Late Permian (254 MYA) to Early Jurassic (176 MYA) [12] . Based on the large number of individual elements counted in some species [13] , it had been suggested that elongation has occurred through the addition of embryonic segments by an increased rate or a prolonged period of somite formation [14] . The homologization of structures is fundamental to understand the mechanism of elongation. In many early actinopterygians, vertebral centra are absent ( Fig. 1d ), and the vertebrae are derived from four separate cartilaginous precursors (arcualia): two dorsal (basidorsal and dorsal intercalary) and two ventral (basiventral and ventral intercalary) [15] ( Fig. 1 ). The basidorsals give rise to the neural arches and spines, and the basiventrals give rise to the haemal arches and spines [16] . Groups thought to be closely related to saurichthyids have either chondrified [17] , [18] or ossified [19] , [20] small, nodular intercalaries. However, no elements corresponding to dorsal intercalaries have been reported in saurichthyids, and it has been proposed that the dorsal intercalaries are enlarged and are indistinguishable from neural arches in these fishes [13] , [21] , [22] . This hypothesis has been met with scepticism [23] . An alternative hypothesis is therefore necessary to explain the alternating morphological pattern of axial elements in some saurichthyids [13] , [21] , [22] , and may involve divergence between successive segments. Here we describe a new specimen of S. curionii (Bellotti, 1857) that, because of its exceptional soft tissue preservation, serves to test the postulated mechanism of elongation. The new fossil originates from the Ladinian (Middle Triassic) Meride Formation of Switzerland, a UNESCO protected fossil site from which rich vertebrate faunas are known, but where preservation of soft tissues is rare. Owing to the exceptional preservation in the abdominal and anterior caudal regions of the body, this discovery permits a definitive assessment of the relationship between the musculature, the underlying skeletal elements and the overlying squamation. When framed in a phylogenetic context, evidence suggests that patterning of the interdorsals as neural arches is a synapomorphy of saurichthyids and represents a novel mechanism for the evolution of elongate body plans in vertebrates. It also supports that patterning of the interventrals as haemal arches occurred after patterning changes in the dorsal axial skeleton. Finally, we suggest that doubling the number of mid-lateral scales to maintain a 1:1 relationship with the number of dorsal arches occurred after the transformation of the dorsal intercalaries into arches, but before the modification of ventral intercalaries into haemal arches. Vertebral morphology in S. curionii In S. curionii, vertebral centra are not ossified, and the right and left halves of the neural and haemal arches are unfused ( Figs 1d and 2 ). In the caudal region, there is a 1:1 relationship between dorsal and ventral elements [24] . 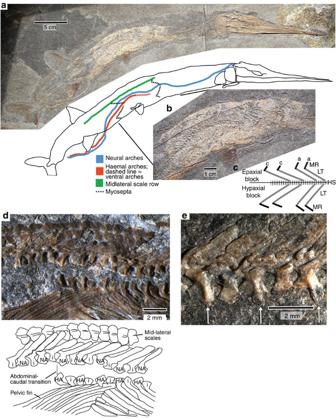Figure 2: Osteology and myology ofS. curionii. (a) PIMUZ T 5806, photo and line drawing with (b) inset showing area of preserved soft tissue, (c) reconstruction of the myosepta with anterior to the right, (d) PIMUZ T 4104, abdominal–caudal transition illustrating vertebral morphology, (e) PIMUZ T 4156, abdominal vertebrae illustrating alternating neural arch morphology with arrows, indicating the true neural arches. a, abdominal myoseptum; c, caudal myoseptum; HA, haemal arch; HS, horizontal septum and flanking multilayer; i, intercalary; LT, lateral tendon; MR, myorhabdoid tendon; and NA, neural arch. Figure 2: Osteology and myology of S. curionii . ( a ) PIMUZ T 5806, photo and line drawing with ( b ) inset showing area of preserved soft tissue, ( c ) reconstruction of the myosepta with anterior to the right, ( d ) PIMUZ T 4104, abdominal–caudal transition illustrating vertebral morphology, ( e ) PIMUZ T 4156, abdominal vertebrae illustrating alternating neural arch morphology with arrows, indicating the true neural arches. a, abdominal myoseptum; c, caudal myoseptum; HA, haemal arch; HS, horizontal septum and flanking multilayer; i, intercalary; LT, lateral tendon; MR, myorhabdoid tendon; and NA, neural arch. Full size image There are two types of dorsal elements distributed in an alternating pattern ( Fig. 2e ). The anterior element (true neural arch, confirmed based on an intermyoseptal position) has a pronounced ridge along the pedicle ( Fig. 2e ). The posterior element (intercalary neural arch) lacks this ridge. As with the neural arches, the haemal arches are distributed in an alternating pattern. The first haemal arch is short and has a strongly developed crest on its posterior margin. All odd-numbered (true) haemal arches show this crest ( Fig. 2d ), whereas it is weakly developed on the even-numbered (intercalary) arches. Axial myology in S. curionii Preserved tendons are observed from the mid-abdominal region to the anterior caudal region ( Fig. 2a–c ). The vertebral column has been ventrally displaced post mortem, so that the horizontal septum and flanking multilayer lies dorsal to the neural arches ( Supplementary Fig. S1 ). The number of segments spanned by a single lateral tendon cannot be determined. In the anteriormost preserved myosepta, the dorsal and ventral posterior myoseptal cones are not preserved. A hypaxial segment is 2.7 mm wide immediately ventral to the horizontal septum; in contrast, a segment defined based on a neural arch is only 1.7 mm wide. The hypaxial lateral tendons (HLT) are anteroposteriorly wider than the epaxial lateral tendons (ELT). Slightly posterior to this initial preserved block of myosepta, the horizontal septum is located at the level of the neural arch pedicles ( Fig. 2a–c ). The dorsal and ventral posterior cones are preserved ( Fig. 2a–c ). The posterior extent of the ventral posterior cone is not significantly greater than the dorsal posterior cone (ELT=11.9 mm; HLT=16.4 mm; the portion of the tendon in the multilayer is omitted in these and subsequent measurements). Epaxial tendons are much thinner and slightly shorter than their hypaxial counterparts ( Fig. 2a–c ). The width of the hypaxial segments increases from 2.7 to 3.7 mm, and the width of the arch-defined segments varies between 1.5 and 1.7 mm. Generally, one tendon is associated with two neural spines, but in some cases, there appears to be a 1:1 relationship between tendons and neural spines. Measurements from the hypaxial block indicate a 2:1 relationship between arches and myosepta, suggesting that some tendons may bifurcate in the epaxial block. In the posteriormost abdominal region, the vertebral column is disarticulated and the epaxial block is not well preserved. In the anterior caudal region, the horizontal septum is displaced ventrally and overlies the base of the haemal arches. Both the dorsal and ventral posterior cones are preserved. These are approximately symmetrical, with the ventral cones being slightly anteroposteriorly longer ( Fig. 2a–c ). There is a 2:1 relationship between the number of haemal arches and myosepta. As in the abdominal region, this ratio is not as clear in the epaxial block. However, because the horizontal septum has been ventrally displaced, it is possible to trace the lateral tendons from the epaxial block ventrally and it is clear that no bifurcation of the tendons occurs. Taphonomy is responsible for the perceived 1:1 relationship between neural spines and ELTs. The myosepta immediately dorsal to the horizontal septum are ~3.4 mm wide. In contrast, an arch-defined segment in this region is ~2.1 mm wide. The lateral tendons are thinner and more elongate than in the abdominal region (ELT=15.2 mm; HLT=20.1 mm). Whereas the HLTs in the abdominal region were anteroposteriorly broad along most of their length, the first two caudal tendons are dorsally broad and rapidly thin ventrally. In more posterior caudal myosepta, the hypaxial tendons are thin along their entire length. In the posterior caudal region, the vertebral column is twisted and displaced. Some posterior myosepta are preserved, but interpretation is difficult. The relationship between myosepta and squamation Rieppel [24] noted that the relationship between the number of neural arches and mid-dorsal scales was 2:1 in S. curionii , whereas the mid-lateral scale row had a 1:1 relationship with the axial elements. We evaluated the relationship between mid-lateral scale row, the myosepta and the vertebral elements in the anterior caudal region, and could confirm a 1:1 relationship between mid-lateral scales and neural arch-like elements, and a 2:1 relationship between scales and myosepta in the anterior caudal region. No morphological differentiation could be detected between alternating scales in the mid-lateral row. Duplication of the neural arches within a somite (by expansion of the intercalaries) represents a novel evolutionary pathway leading to axial elongation, and incorporates aspects of both somitic elongation and high meristic counts ( Fig. 1c ). Dorsal arch counts in saurichthyids range from 136 to 210 ( S. curionii : 170–180 (ref. 24 ), and therefore axial somite counts range from 68 to 105 ( S. curionii : 85–90). This is in the range of some closely related fishes lacking an elongate body plan: Birgeria groenlandica and B. stensioei have counts of at least 80 and 89, respectively [20] . When mapped on the phylogenetic topology ( Fig. 3 ), there is no evidence of a large increase in the number of somites between Saurichthyidae and Birgeria (contra Schmid [14] , who counted each neural arch-like structure as a separate segment in Saurichthys ). Although this is the first instance of two neural arch-like segments reported in vertebrates, diplospondyly (two mineralized vertebral centra per segment) is relatively widespread among fishes [16] , [25] and is thought to increase flexibility of the vertebral column [26] . Axial flexibility in saurichthyids will be discussed in more detail below; however, a perceived trend towards features increasing the stability of the axial skeleton in these fishes [12] , [27] suggests functional differences from diplospondyly. 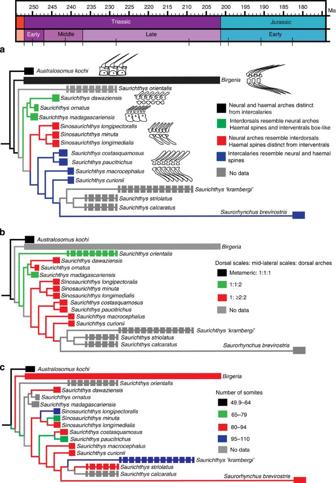Figure 3: Mapping the evolution of morphological characters on a saurichthyid phylogeny. (a) Evolution of the neural arches, interdorsals, haemal arches and interventrals, (b) evolution of the mid-dorsal and mid-lateral scales, and dorsal vertebral elements (neural spines+expanded intercalaries), (c), number of somites reconstructed using squared-change parsimony. Timescale produced with TSCreator (http://tscreator.org), see Methods for information regarding the phylogenetic hypothesis. Vertebral morphology modified from refs13,19,20,21,22,24. Figure 3: Mapping the evolution of morphological characters on a saurichthyid phylogeny. ( a ) Evolution of the neural arches, interdorsals, haemal arches and interventrals, ( b ) evolution of the mid-dorsal and mid-lateral scales, and dorsal vertebral elements (neural spines+expanded intercalaries), ( c ), number of somites reconstructed using squared-change parsimony. Timescale produced with TSCreator ( http://tscreator.org ), see Methods for information regarding the phylogenetic hypothesis. Vertebral morphology modified from refs 13 , 19 , 20 , 21 , 22 , 24 . Full size image Expansion of the intercalaries such that they are virtually indistinguishable from the neural and haemal arches is conclusively demonstrated in S. curionii based on the exceptional preservation of soft tissue, which provides information on the width and position of myosepta (reconstructed in Fig. 4 ). The alternative hypothesis, that alternating vertebral segments vary in morphology, can be rejected. Previously undescribed osteological differences are present between successive elements, and restudy indicates that these differences are also present in other species in which myoseptal information is not directly available ( S. costasquamosus, S. paucitrichus, S. macrocephalus and Saurorhynchus brevirostris ). When similarity between the neural arches and intercalaries is mapped over the new species-level topology ( Fig. 3a ), it becomes clear that two neural arch-like structures per segment is likely a synapomorphy of saurichythyids [13] . Saurichthyids thus represent the first known exception to the rule that all neural arch-like structures are intersegmental in position [28] , and suggests that intercalaries can develop a complex morphology and be conserved over long evolutionary time spans (contra Bartsch and Gemballa [29] and Laerm [30] ). 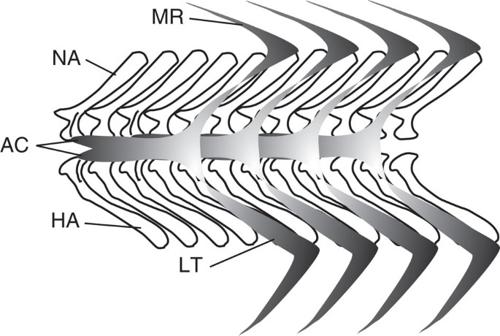Figure 4: Reconstruction of the myosepta inSaurichthys. Hypothesized relationship between skeletal elements and myoseptal tendons in the anterior caudal region ofSaurichthys, assuming that the anterior cone spans three myomeric segments. Anterior is to the left. AC, anterior cone; HA, haemal arch; LT, lateral tendon; MR, myorhabdoid tendon; and NA, neural arch. Figure 4: Reconstruction of the myosepta in Saurichthys . Hypothesized relationship between skeletal elements and myoseptal tendons in the anterior caudal region of Saurichthys , assuming that the anterior cone spans three myomeric segments. Anterior is to the left. AC, anterior cone; HA, haemal arch; LT, lateral tendon; MR, myorhabdoid tendon; and NA, neural arch. Full size image Morphological differentiation between the haemal arches and ventral intercalaries is retained in many Lower and Middle Triassic saurichthyids ( Fig. 3a ), unlike the situation in the dorsal vertebral column [13] , [21] , [23] . A 1:1 relationship between dorsal elements bearing neural spines and ventral elements bearing haemal spines arose secondarily in the European species of Middle Triassic age and younger [24] , [31] , [32] . Thus, it seems probable that the expansion of the dorsal and ventral intercalaries occurred independently, with the change in the former preceding that in the latter. In extant actinopterygians bracketing the hypothesized phylogenetic position of Saurichthys (that is, Lepisosteus and Polypterus ), a 1:1 relationship exists between myomeres and ganoid scale rows [33] , [34] . Metameric squamation, one scale row per vertebral segment, has also been noted in the Triassic genus Australosomus [20] , used as the outgroup in our analysis. Other forms of a similar grade (for example, Boreosomus [35] , [36] ) show polymeric squamation [37] , in which many scales are present per vertebral segment, making polarization of this character uncertain. However, the 1:1:2 relationship between scales of the mid-dorsal row, mid-lateral row and neural arch-like elements found in basal saurichthyids (for example, S. orientalis and S. madagascariensis ) [23] , [38] , [39] suggests that a metameric pattern of squamation was plesiomorphic for the family, and metameric squamation persisted following expansion of the interdorsals ( Fig. 3b ). The 1:1 relationship between the mid-lateral scales and neural arch-like elements, thus a 1:2 relationship between mid-lateral scales and somites, observed in the European Middle Triassic species arose later. Similarities between the number of dorsal arch elements and the squamation, rather than between the myosepta and the squamation, may have had implications for lateral bending of the body. The preserved myosepta of S. curionii provide information on the functional implications of axial elongation by duplication of neural arches within a somite. The length of the lateral tendon can approximate swimming style in living chondrichthyans and actinopterygians [9] . Carangiform and thunniform swimmers are characterized by much longer lateral tendons in the caudal region than in the abdominal region, up to 15–25% total length (TL) [9] , [40] , [41] . Caudal tendons of 6–10% TL, only slightly longer than the abdominal tendons, characterize anguilliform to sub-carangiform swimmers [9] , [40] , [41] , [42] , [43] , and extremely flexible fishes show caudal tendons shorter or equal to abdominal tendons in length and <5% TL [42] , [43] . In S. curionii, the length of a hypaxial myoseptum is 5.1% TL in the abdominal region and 6.4% TL in the caudal region. These values are minimal approximations because most of the variation in the numerator—tendon length—is found in the anterior myoseptal cone [9] , which cannot be measured in Saurichthys , and the denominator is increased because of the disproportionately elongate skull in S. curionii. These values are similar to those obtained from a range of sub-carangiform to anguilliform swimmers, including non-teleost actinopterygians [9] , but are inconsistent with both highly flexible fishes [42] , [43] and carangiform to thunniform swimmers [9] . Although both an unconstricted notochord and an increased number of axial elements—and therefore joints—in the skeleton are associated with greater axial flexibility [5] , [44] , [45] , the myoseptal morphology of Saurichthys is inconsistent with this inference. Geological and ecological data suggest that S. curionii was associated with a carbonate platform environment [24] , [32] , [46] , and some morphological cues such as body outline and reduced squamation [12] , [47] are inferred to be related to good acceleration performance constrained by piscivory [48] , [49] , [50] , [51] . Dietary inferences are supported by stomach contents [24] . Although fishes occupying this niche typically have an elongate body shape, they do not usually show extreme axial flexibility [52] , [53] , [54] . We present the first report of elongation of the axial skeleton by within-segment element duplication in a vertebrate. This unique mechanism is associated with the greater disparity in vertebral morphology and development in non-teleostean actinopterygians than in teleosts [28] . The soft tissue preservation in the described fossil specimen provides definitive evidence on element homology supporting this conclusion, as well as an understanding of the elongation process and a clarification of some aspects of locomotion. Tendon morphology indicates that S. curionii does not show specializations for active pelagic swimming nor for high axial flexibility. Increasing the number of dorsal arches without an increase in the number of myomeres may be a biomechanical compromise, enhancing the stability of a poorly ossified vertebral column in an elongate body without increasing axial flexibility. This unique innovation may be responsible for the enormous success of saurichthyid fishes in the Early and Middle Triassic [12] . Specimen description The specimen PIMUZ (Paläontologisches Institut und Museum, Universität Zürich) T 5806 ( Fig. 2a ) was excavated in 1975 by the PIMUZ from the Cassina Member of the Lower Meride Formation (240.63±0.13 MYA; Ladinian [55] ) at the Cassina locality. Some disruption of the axial skeleton has occurred, but this did not affect the lateral structures on the right side. The soft tissue structures preserved on PIMUZ T 5806 are myoseptal tendons rather than myomeres. Tendons are more resistant to decay than muscle tissue due to higher collagen content [56] , and, in addition, the structures are dorsally and ventrally narrow and show limited overlap, which is more consistent with tendons than myomeres. PIMUZ T 5806 is referred to S. curionii based on its gracile rostrum, reduced dentition, shape of the operculum, pattern of squamation and stratigraphic provenance [24] , [32] , [57] . The specimen has a TL of 517 mm, which lies outside the published size range for this species [24] . Vertebral morphology is difficult to assess because of the overlying soft tissue. For that reason, we rely on additional complete or nearly complete specimens of S. curionii from the PIMUZ collection to evaluate skeletal morphology (PIMUZ T3913, T 3914, T 3917, T 4104, T 4105, T 4156, T 5638, T 5657 and T 5679). We use the terminology of Sallan [11] to refer to ventral ossifications anterior and posterior to the abdominal–caudal transition, and the terminology of Gemballa et al . [58] for myoseptal tendons. To compare tendon lengths in Saurichthys to extant fishes, we added the length of six dorsal arches to the length of the lateral tendon, because in most actinopterygians, including those without ossified vertebral centra (for example,, Acipenser ), the lateral tendons extend horizontally over a minimum of three vertebrae [33] . We then divided this tendon length estimate by TL. Phylogenetic analysis Only a single previous study examined ingroup relationships of saurichthyid fishes [32] . To frame our results in a phylogenetic context, we expanded this analysis to 17 species and 52 characters coded from the literature and study of specimens in museum collections ( Supplementary Notes 1 and 2 ). Nine characters derived from the division of count or shape continua were treated as ordered. Data were analysed in Tree analysis using New Technology (TNT) [59] using the implicit enumeration search option and a maximum parsimony optimization criterion. This resulted in a single most parsimonious tree (length 132 steps, consistency index (CI)=0.52). Characters relating to axial morphology and squamation were reconstructed on the resulting topology ( Fig. 3 ). These characters were also included in the generation of the tree topology, thus, these characters are not an independent data source. To determine whether there was an increase in the number of somites in Saurichthyidae, independent of other mechanisms, we plotted the total number of vertebrae over phylogeny using weighted squared-change parsimony implemented in Mesquite [60] ( Fig. 3 ). Branch lengths were constrained using the earliest occurrence of the terminal taxa. Total numbers of vertebrae for species were taken from counts obtained firsthand from museum specimens (EM) or the literature [13] , [20] , [22] , [24] . How to cite this article: Maxwell, E. E. et al . Exceptional fossil preservation demonstrates a new mode of axial skeleton elongation in early ray-finned fishes. Nat. Commun. 4:2570 doi: 10.1038/ncomms3570 (2013).